Correspondence: Space-time asymmetry undermines water yield assessment 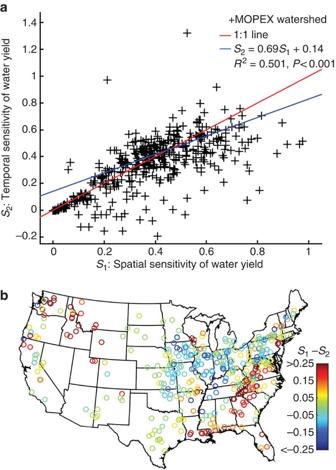Figure 1: Spatial and temporal sensitivity of water yield. Spatial sensitivity of water yield (x-axis) and temporal sensitivity of water yield (y-axis) for 420 watersheds located in the United States (a), and the spatial pattern of their differences (b). Water yield sensitivity calculations Zhou et al . [1] used the partial derivative of Fuh’s equation to calculate the water yield sensitivity to wetness index: where P , PET and m denote the long-term average values of precipitation, potential evaporation and watershed characteristics. We calculate water yield sensitivity to climate based on temporal differences using the slope ( α ): where is the water yield of year i , and is the wetness index of year i . The α value is approximated by the slope terms of least-squares estimators. Annual values used in the analysis are from 1 September to 31 August to minimize the effects of carry-over of water storage. Repeating the analysis for 5-year values yields similar results. How to cite this article: Berghuijs, W. R. & Woods, R. A. Correspondence: Space-time asymmetry undermines water yield assessment. Nat. Commun. 7:11603 doi: 10.1038/ncomms11603 (2016).